A functional interaction between Hippo-YAP signalling and FoxO1 mediates the oxidative stress response The Hippo pathway is an evolutionarily conserved regulator of organ size and tumorigenesis that negatively regulates cell growth and survival. Here we report that Yes-associated protein (YAP), the terminal effector of the Hippo pathway, interacts with FoxO1 in the nucleus of cardiomyocytes, thereby promoting survival. YAP and FoxO1 form a functional complex on the promoters of the catalase and manganese superoxide dismutase (MnSOD) antioxidant genes and stimulate their transcription. Inactivation of YAP, induced by Hippo activation, suppresses FoxO1 activity and decreases antioxidant gene expression, suggesting that Hippo signalling modulates the FoxO1-mediated antioxidant response. In the setting of ischaemia/reperfusion (I/R) in the heart, activation of Hippo antagonizes YAP-FoxO1, leading to enhanced oxidative stress-induced cell death through downregulation of catalase and MnSOD. Conversely, restoration of YAP activity protects against I/R injury. These results suggest that YAP is a nuclear co-factor of FoxO1 and that the Hippo pathway negatively affects cardiomyocyte survival by inhibiting the function of YAP-FoxO1. Originally identified in Drosophila melanogaster , the Hippo pathway is an evolutionarily conserved regulator of organ size that controls both cell proliferation and apoptosis [1] . The key components of the mammalian Hippo pathway include sterile 20-like kinases (Mst1 and Mst2; homologues of D. hippo ), the large tumour suppressors (Lats1 and Lats2; homologues of warts ) and Yes-associated protein (YAP) and its paralog protein transcriptional co-activator with PDZ-binding motif (TAZ), transcriptional co-activators and homologues of yorkie . YAP/TAZ regulates the transcriptional activity of TEA domain family (TEAD), p73 and Runx2 in the nucleus, thereby controlling growth and death in many cell types [1] . Activation of Lats1/2 by Mst1/2 induces phosphorylation and nuclear exit/proteolytic degradation of YAP/TAZ, thereby negatively regulating YAP/TAZ. Increasing lines of evidence suggest that inactivation of the Hippo pathway leads to uncontrolled cell proliferation in epithelial cells and stem cells [2] , [3] and oncogenic transformation [4] , [5] , [6] , both of which are mediated through hyperactivity of YAP [2] , [3] . Hippo signalling and its regulation of YAP modulate heart size by restraining cardiomyocyte proliferation during fetal development [7] , [8] . Recent evidence suggests that activation of YAP also promotes myocardial regeneration after myocardial infarction by promoting proliferation of cardiomyocytes in adult hearts [9] , whereas activation of the Hippo components, including Mst1 and/or Lats2, in the adult heart promotes cardiomyocyte apoptosis [10] , [11] . Postnatal genetic deletion of YAP leads to cardiac dysfunction and premature death in mice [12] , suggesting that the upstream Hippo pathway promotes cell death and that YAP promotes cell survival in post-mitotic hearts. It should be noted that the molecular mechanism through which YAP promotes cell survival in cardiomyocytes is unknown. Given that YAP acts as a transcriptional co-factor, it is important to identify the transcription factor(s) through which YAP promotes cardiomyocyte survival in postnatal hearts. The Hippo signalling pathway has an important role in mediating oxidative stress-induced cell death. For example, Mst1 mediates neuronal cell death in response to H 2 O 2 (ref. 13 ). Ischaemia/reperfusion (I/R), which is known to cause myocardial injury and cardiac dysfunction, induces enhanced production of reactive oxygen species (ROS) and cardiomyocyte death through Mst1-dependent mechanisms [10] . Interestingly, stimulation of YAP prevents, whereas downregulation of YAP promotes, H 2 O 2 -induced cardiomyocyte death [12] , suggesting causative involvement of YAP in cardiomyocyte survival during oxidative stress. However, the molecular mechanism through which YAP mediates the survival of cardiomyocytes remains to be elucidated. FoxO1 belongs to the family of transcription factors possessing a conserved DNA-binding domain termed as the ‘Forkhead box’ [14] . FoxO1 has a fundamental role in regulating cell cycle, apoptosis, atrophy, autophagy and energy homeostasis [14] , [15] . FoxO1 also mediates protective effects against oxidative stress through regulation of antioxidant genes including catalase and MnSOD [16] , [17] . Conditional deletion of FoxO1 in the heart increases cell death and reduces cardiac function in response to myocardial infarction, suggesting that FoxO1 promotes cardiomyocyte survival in response to oxidative stimuli [18] . However, the signalling cascade that regulates FoxO1 activity during I/R is not yet understood. Here we show that YAP forms a functional complex with FoxO1 in mediating antioxidant gene expression in response to I/R in the heart. Activation of Hippo signalling inhibits the YAP-FoxO1 complex and promotes cell death in response to oxidative stress. Our results suggest that FoxO1 acts as a downstream effector of YAP to regulate cardiomyocyte survival. YAP functions as a transcriptional co-activator of FoxO1 We have shown previously that downregulation of YAP confers cellular hypersensitivity to ROS and induces cardiomyocyte death in vitro [12] . Consistently, cardiac-specific deletion of YAP induced accumulation of ROS in the mouse heart ( Supplementary Fig. 1a,b ), suggesting that YAP is involved in redox homeostasis regulation. FoxO1 transcriptionally upregulates antioxidant genes in response to oxidative stress and prevents cell death [16] , [17] . Given the fact that Hippo-YAP signalling mediates cell death in response to oxidative stress, we hypothesized that FoxO1 may functionally interact with the Hippo pathway. We performed immunocytochemistry experiments and found that YAP and FoxO1 co-localized in the nucleus ( Fig. 1a ). Using the in situ proximity ligation assay, we also observed that endogenous YAP and FoxO1 physically interact with one another in the nuclei of neonatal cardiomyocytes in vitro and adult cardiomyocytes in the mouse heart in vivo ( Fig. 1b and Supplementary Fig. 2a ). Co-immunoprecipitation assays confirmed that endogenous YAP associates with FoxO1 in cardiomyocytes ( Fig. 1c ), and glutathione S -transferase (GST) pull-down assays revealed that YAP directly binds to FoxO1 ( Fig. 1d ). YAP dose-dependently stimulated FoxO1 transcriptional activity, as evaluated with a FoxO1-luciferase reporter gene (FoxO1-luc) driven by three canonical FoxO1-response elements ( Fig. 1e ). Taken together, these results suggest that YAP acts as a transcriptional co-activator of FoxO1. As FoxO1 and FoxO3 have overlapping functions in the heart, we examined whether YAP also interacts with FoxO3. Co-immunoprecipitation assays showed that YAP was not associated with FoxO3 ( Supplementary Fig. 2b ), indicating isoform-specific interaction between YAP and FoxO1. We further examined which domain of YAP is essential for physical interaction with and transcriptional activation of FoxO1. Mutation of Ser 94 in the TEAD-binding site to alanine (S94A) significantly reduced the interaction between YAP and FoxO1, and partially attenuated YAP-mediated FoxO1 activation ( Supplementary Fig. 2c,d ). Although N-terminal YAP, lacking the transcriptional activation domain located in the C-terminal, did not affect YAP binding ( Supplementary Fig. 2c ), it also attenuated YAP-mediated FoxO1 activation ( Supplementary Fig. 2d ). On the other hand, deletion of the WW domain in YAP (ΔWW) affected neither FoxO1 binding nor YAP-mediated FoxO1 activation ( Supplementary Fig. 2c,d ). Taken together, these results indicate that both the TEAD-binding site and the C-terminal transactivation domain of YAP are important for YAP-mediated FoxO1 activation. 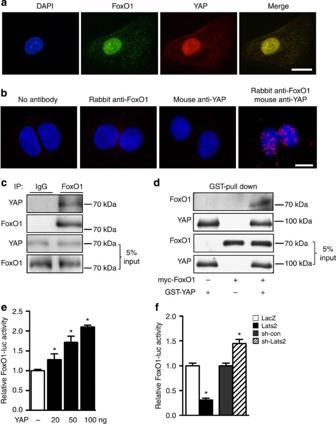Figure 1: YAP interacts with FoxO1 and regulates its transcriptional activity. (a) The localization of FoxO1 and YAP was examined. Myocytes were stained with FoxO1 (red), YAP (green) and DAPI (blue). Scale bar, 10 μm. (b) Cells were stained with Rabbit anti-FoxO1 antibody and/or Mouse anti-YAP antibody, andin vivoprotein–protein interaction between FoxO1 and YAP (red dots) was detected with secondary proximity probes, anti-Rabbit-PLUS and anti-Mouse-MINUS, using the Duolinkin situPLA detection kit. Scale bar, 10 μm. (c) Neonatal cardiomyocyte lysates were prepared and immunoprecipitated with FoxO1 antibody or control IgG. The interaction between FoxO1 and YAP was examined. Immunoblots of input lysate controls (5% of inputs) are also shown. (d) Recombinant GST-YAP and myc-FoxO1 were used to examine the direct interaction between YAP and FoxO1. (e) Cardiomyocytes were co-transfected with 1 μg FoxO1-luc vector and the indicated expression vectors. After 48 h, the luciferase activity was measured, demonstrating that YAP enhanced FoxO1 transcriptional activity (*P<0.05 versus empty vector,n=3). (f) Overexpression of Lats2 inhibited, whereas knockdown of Lats2 enhanced, FoxO1 activity. Cardiomyocytes were transfected with 1 μg FoxO1-luc vector. After 6 h, myocytes were transduced with the indicated virus and luciferase activity was measured (*P<0.05 versus LacZ or sh-con,n=3). Data are shown as mean±s.e.m.Pvalues were determined using unpaired Student’st-test. Figure 1: YAP interacts with FoxO1 and regulates its transcriptional activity. ( a ) The localization of FoxO1 and YAP was examined. Myocytes were stained with FoxO1 (red), YAP (green) and DAPI (blue). Scale bar, 10 μm. ( b ) Cells were stained with Rabbit anti-FoxO1 antibody and/or Mouse anti-YAP antibody, and in vivo protein–protein interaction between FoxO1 and YAP (red dots) was detected with secondary proximity probes, anti-Rabbit-PLUS and anti-Mouse-MINUS, using the Duolink in situ PLA detection kit. Scale bar, 10 μm. ( c ) Neonatal cardiomyocyte lysates were prepared and immunoprecipitated with FoxO1 antibody or control IgG. The interaction between FoxO1 and YAP was examined. Immunoblots of input lysate controls (5% of inputs) are also shown. ( d ) Recombinant GST-YAP and myc-FoxO1 were used to examine the direct interaction between YAP and FoxO1. ( e ) Cardiomyocytes were co-transfected with 1 μg FoxO1-luc vector and the indicated expression vectors. After 48 h, the luciferase activity was measured, demonstrating that YAP enhanced FoxO1 transcriptional activity (* P <0.05 versus empty vector, n =3). ( f ) Overexpression of Lats2 inhibited, whereas knockdown of Lats2 enhanced, FoxO1 activity. Cardiomyocytes were transfected with 1 μg FoxO1-luc vector. After 6 h, myocytes were transduced with the indicated virus and luciferase activity was measured (* P <0.05 versus LacZ or sh-con, n =3). Data are shown as mean±s.e.m. P values were determined using unpaired Student’s t -test. Full size image Lats2-YAP axis regulates FoxO1 activity Phosphorylation of YAP at Ser 127 by Lats2 promotes nuclear exclusion and cytoplasmic accumulation of YAP, thereby leading to its inactivation [19] . In order to examine whether the Hippo signalling pathway regulates FoxO1 through a YAP-dependent mechanism, we overexpressed either Mst1 or Lats2 in cardiomyocytes, as activation of either Mst1 or Lats2 induces a strong Hippo phenotype in the heart [10] , [11] , namely promotion of cardiomyocyte apoptosis and suppression of compensatory hypertrophy. Overexpression of Mst1 enhanced the phosphorylation of Ser 872 and Thr 1041 of Lats2, indicating full activation of Lats2 (ref. 20 ), as well as Ser 127 phosphorylation of YAP ( Supplementary Fig. 3a ). Lats2 was mainly localized in the nucleus ( Supplementary Fig. 3b,c ) and overexpression of Lats2 induced nuclear exclusion of YAP ( Supplementary Fig. 3d ), suggesting that Lats2 activation is sufficient to suppress YAP activity in cardiomyocytes. Luciferase assays revealed that overexpression of Lats2 inhibited, whereas downregulation of Lats2 enhanced, the transcriptional activity of FoxO1 ( Fig. 1f ). The transcriptional activity of FoxO1 is primarily dependent upon the phosphorylation status of multiple amino-acid residues [14] . To rule out the possibility that Lats2 regulates FoxO1 activity through direct phosphorylation, an in vitro kinase assay was performed using myc-tagged FoxO1 as a substrate. We observed that FoxO1 was not phosphorylated in the presence of a constitutively active form of Lats2 ( Supplementary Fig. 4a ). Importantly, downregulation of YAP completely abolished the increase in FoxO1 transcriptional activity observed in the presence of Lats2 knockdown alone ( Supplementary Fig. 4b,c ). Therefore, these data suggest that the transcriptional activity of FoxO1 is regulated by the Lats2-YAP axis. As phosphorylation of FoxO1 at Thr 24 and Ser 256 by Akt induces 14-3-3 binding and cytosolic translocation of FoxO1 (refs 21 , 22 ), we next examined whether transcriptional inactivation of FoxO1 induced by Lats2 activation is mediated by Akt. In cardiomyocytes, overexpression of Lats2 affected neither the activity of Akt, as evaluated by its Ser 473 phosphorylation level, nor the level of FoxO1 phosphorylation at Thr 24 and Ser 256 ( Supplementary Fig. 4d ). Although overexpression of YAP induced Akt activation, we did not observe significant changes in phosphorylated FoxO1 levels ( Supplementary Fig. 4e ), indicating that Hippo signalling regulates FoxO1 through Akt-independent mechanisms. The YAP-FoxO1 complex mediates antioxidant gene expression In order to examine whether YAP is involved in FoxO1-mediated antioxidant gene expression, chromatin immunoprecipitation (ChIP) was performed using FoxO1 and YAP antibodies in H9C2 myoblast cells. Mapping of the promoter regions of catalase and MnSOD indicated that each promoter has two conserved FoxO1-binding motifs ( Fig. 2a ), both of which are required for FoxO1 binding and transcriptional activation in response to oxidative stress [16] , [17] . After ChIP with YAP antibody, primer sets designed to detect the FoxO1 DNA-binding sites in both promoters were used for PCR analysis. These experiments revealed that YAP was present at the FoxO1-binding motifs in the promoter regions of both catalase and MnSOD ( Fig. 2b ). As expected, ChIP with FoxO1 antibody showed that FoxO1 binds to the same regions. In order to confirm that YAP is co-localized with FoxO1 on the promoters of catalase and MnSOD, sequential ChIPs were conducted. The first ChIP was performed with FoxO1 antibody and the second ChIP was carried out with either YAP or FoxO1 antibody using the chromatin eluted from the first ChIP. Following the second ChIP, both YAP and FoxO1 were still bound to the FoxO1-binding motifs in the FoxO1–chromatin complex ( Fig. 2b ), confirming that YAP and FoxO1 are present at the same promoter regions of catalase and MnSOD. In order to examine whether YAP and FoxO1 form a functional complex to regulate antioxidant gene expression, a luciferase vector was generated that contained a minimal promoter region of catalase (catalase-luc), including one FoxO1 DNA-binding site close to the transcriptional start site. Co-transfection of FoxO1 with catalase-luc enhanced the luciferase activity, but this enhancement was completely abolished by YAP knockdown. Co-transfection of YAP with catalase-luc also caused enhanced luciferase activity, which was completely abolished by FoxO1 depletion ( Fig. 2c ). These results indicate that YAP is an essential co-factor of FoxO1 and is required to maintain its transcriptional activation of antioxidant gene expression. 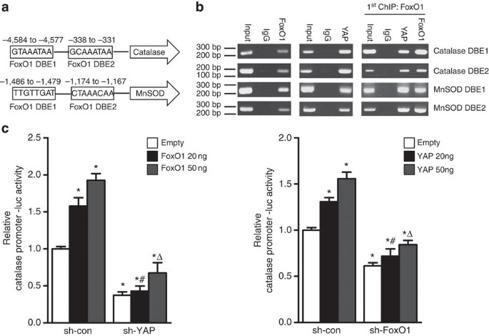Figure 2: YAP is essential for FoxO1-mediated antioxidant gene expression. (a) The catalase and MnSOD promoters contain two potential FoxO1 DNA-binding elements referred to as DBE1 and DBE2. (b) ChIP analysis ofin vivoYAP and FoxO1 binding to the catalase and MnSOD promoters. Protein-bound chromatin was prepared from H9C2 myoblasts and immunoprecipitated with YAP or FoxO1 antibodies. For sequential ChIP, the protein-bound chromatin was first immunoprecipitated with the FoxO1 antibody. The second ChIP was then performed on the chromatin eluted from the first ChIP by immunoprecipitating it with the YAP antibody. Normal IgG was used as a negative control. The immunoprecipitated DNA was analysed by PCR using primers flanking each of the DBEs. Results are representative of three individual experiments. (c) The minimal catalase promoter containing FoxO1 DBE2 was cloned into a luciferase vector. Cardiomyocytes were co-transfected with the catalase-luc vector and the indicated expression vectors. After 6 h, myocytes were transduced with the indicated virus and, after 72 h, the luciferase activity was measured (*P<0.05 versus empty vector, #P<0.05 versus 20 ng FoxO1 or YAP, ΔP<0.05 versus 50 ng FoxO1 or YAP,n=3). Data are shown as mean±s.e.m..Pvalues were determined using one-way ANOVA followed by a Newman–Keuls comparison test. Figure 2: YAP is essential for FoxO1-mediated antioxidant gene expression. ( a ) The catalase and MnSOD promoters contain two potential FoxO1 DNA-binding elements referred to as DBE1 and DBE2. ( b ) ChIP analysis of in vivo YAP and FoxO1 binding to the catalase and MnSOD promoters. Protein-bound chromatin was prepared from H9C2 myoblasts and immunoprecipitated with YAP or FoxO1 antibodies. For sequential ChIP, the protein-bound chromatin was first immunoprecipitated with the FoxO1 antibody. The second ChIP was then performed on the chromatin eluted from the first ChIP by immunoprecipitating it with the YAP antibody. Normal IgG was used as a negative control. The immunoprecipitated DNA was analysed by PCR using primers flanking each of the DBEs. Results are representative of three individual experiments. ( c ) The minimal catalase promoter containing FoxO1 DBE2 was cloned into a luciferase vector. Cardiomyocytes were co-transfected with the catalase-luc vector and the indicated expression vectors. After 6 h, myocytes were transduced with the indicated virus and, after 72 h, the luciferase activity was measured (* P <0.05 versus empty vector, # P <0.05 versus 20 ng FoxO1 or YAP, Δ P <0.05 versus 50 ng FoxO1 or YAP, n =3). Data are shown as mean±s.e.m.. P values were determined using one-way ANOVA followed by a Newman–Keuls comparison test. Full size image Hippo signalling suppresses antioxidant gene expression We next examined the role of the Hippo signalling pathway in the regulation of catalase and MnSOD expression in intact cells, as overexpression of Lats2 is sufficient to suppress FoxO1-mediated transcription ( Fig. 1f ). ChIP assays revealed that overexpression of Lats2 significantly reduced the amount of YAP present at the FoxO1-binding sites in the promoter regions of catalase and MnSOD ( Fig. 3a ). Furthermore, the mRNA and protein levels of both catalase and MnSOD were decreased by Lats2 overexpression ( Fig. 3b,c ). On the other hand, downregulation of Lats2 increased both the mRNA and protein levels of catalase and MnSOD ( Fig. 3b,c ). The enhancement in catalase-luc activity observed in Lats2 knockdown cells was completely reversed by simultaneous downregulation of either YAP or FoxO1 ( Fig. 3d ). These data indicate that the Lats2-YAP-FoxO1 nexus is essential for regulating expression of these antioxidant enzymes. Both catalase and MnSOD can effectively convert superoxide and hydrogen peroxide to water in order to prevent ROS accumulation and protect against cell death from oxidative stress. Inhibition of Lats2 reduced myocyte death in response to H 2 O 2 treatment, but not when the cells were co-transduced with adenovirus harbouring FoxO1 short hairpin RNA (ad-sh-FoxO1) or YAP short hairpin RNA (ad-sh-YAP) ( Fig. 3e and Supplementary Fig. 4f ), suggesting that Lats2 activation impairs the antioxidant defence and triggers cell death through suppression of YAP-FoxO1. Taken together, these data suggest a novel mechanism in which Hippo signalling activation regulates cell death through suppression of the FoxO1-mediated antioxidant response during oxidative stress. 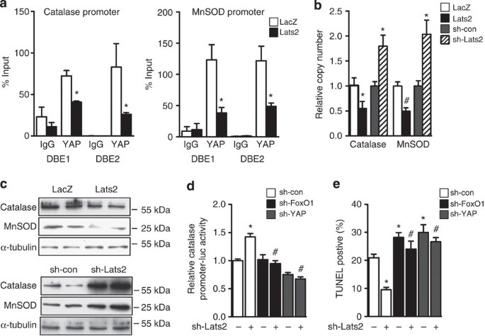Figure 3: Hippo activation promotes cell death in response to oxidative stress. (a) ChIP analysis ofin vivoYAP binding to the catalase and MnSOD promoters. H9C2 myoblasts were transduced with the indicated adenovirus for 48 h. Protein-bound chromatin was prepared and immunoprecipitated with IgG and YAP antibodies. The relative occupancy on the promoters was compared with the input signal (*P<0.05 versus LacZ,n=3). (b,c) Overexpression of Lats2 reduced, whereas knockdown of Lats2 enhanced, catalase and MnSOD protein and mRNA levels. Cardiomyocytes were transduced with the indicated adenovirus. (b) The mRNA levels of catalase and MnSOD were examined by quantitative RT–PCR. The relative copy number was normalized with β-actin (*P<0.05 versus LacZ or sh-con, #P<0.01 versus LacZ,n=4). (c) Lysates were used for immunoblot analysis of catalase, MnSOD and α-tubulin. Results are representative of three individual experiments. (d) Cardiomyocytes were transfected with the catalase-luc vector. After 6 h, myocytes were transduced with the indicated virus and, after 72 h, luciferase activity was measured (*P<0.05 versus sh-con/sh-Lats2(−), #P<0.05 versus sh-con/sh-Lats2(+),n=3). (e) Downregulation of Lats2 prevented H2O2-induced cell death. Cardiomyocytes transduced with the indicated adenovirus were treated with 100 μM H2O2, and TUNEL-positive cells were examined (*P<0.05 versus sh-con/sh-Lats2(−), #P<0.05 versus sh-con/sh-Lats2(+),n=4). Data are shown as mean±s.e.m.Pvalues were determined using unpaired Student’st-test or one-way ANOVA followed by a Newman–Keuls comparison test. Figure 3: Hippo activation promotes cell death in response to oxidative stress. ( a ) ChIP analysis of in vivo YAP binding to the catalase and MnSOD promoters. H9C2 myoblasts were transduced with the indicated adenovirus for 48 h. Protein-bound chromatin was prepared and immunoprecipitated with IgG and YAP antibodies. The relative occupancy on the promoters was compared with the input signal (* P <0.05 versus LacZ, n =3). ( b , c ) Overexpression of Lats2 reduced, whereas knockdown of Lats2 enhanced, catalase and MnSOD protein and mRNA levels. Cardiomyocytes were transduced with the indicated adenovirus. ( b ) The mRNA levels of catalase and MnSOD were examined by quantitative RT–PCR. The relative copy number was normalized with β-actin (* P <0.05 versus LacZ or sh-con, # P <0.01 versus LacZ, n =4). ( c ) Lysates were used for immunoblot analysis of catalase, MnSOD and α-tubulin. Results are representative of three individual experiments. ( d ) Cardiomyocytes were transfected with the catalase-luc vector. After 6 h, myocytes were transduced with the indicated virus and, after 72 h, luciferase activity was measured (* P <0.05 versus sh-con/sh-Lats2(−), # P <0.05 versus sh-con/sh-Lats2(+), n =3). ( e ) Downregulation of Lats2 prevented H 2 O 2 -induced cell death. Cardiomyocytes transduced with the indicated adenovirus were treated with 100 μM H 2 O 2 , and TUNEL-positive cells were examined (* P <0.05 versus sh-con/sh-Lats2(−), # P <0.05 versus sh-con/sh-Lats2(+), n =4). Data are shown as mean±s.e.m. P values were determined using unpaired Student’s t -test or one-way ANOVA followed by a Newman–Keuls comparison test. Full size image Hippo activation enhances oxidative stress in vivo We next sought to further assess the physiological implications of our observations. Reperfusion injury occurs when the blood supply resumes after a period of ischaemia and causes cell death and dysfunction in critical organs, including the heart and the brain [23] . Reperfusion injury is caused primarily by oxidative stress [23] . Inactivation of the upstream Hippo pathway kinase, Mst1, has been shown to reduce I/R injury in the heart and attenuate neuron cell death [10] , [13] . Immunoblot results revealed that I/R strongly induces phosphorylation of Mst1, Lats2 and YAP ( Fig. 4a ), suggesting that Hippo signalling is activated during I/R in the heart. Increased phosphorylation of YAP at Ser 127 and decreased YAP abundance in the nuclear fraction were observed in wild-type (WT) mice after I/R, effects of which were completely attenuated in dominant-negative lats2 (Tg-DN-Lats2) transgenic mice ( Fig. 4a,b ), in which Lats2 kinase activity is completely suppressed [11] , suggesting that endogenous Lats2 mediates Ser 127 phosphorylation and inactivation of YAP in response to I/R. The protein levels of catalase and MnSOD were significantly decreased in WT mice but not in Tg-DN-Lats2, indicating that Hippo activation decreased antioxidant gene expression during I/R in vivo ( Fig. 4c ). The global antioxidant capacity of heart homogenates after I/R was also dramatically decreased in WT mice but not in Tg-DN-Lats2 mice ( Fig. 4d ). We further investigated the extent of oxidative stress-induced damage during I/R. Tissue samples were stained with anti-8-hydroxy-2′-deoxyguanosine (8-OHdG) antibody, a marker of oxidative DNA damage. Immunohistochemistry results revealed that Tg-DN-Lats2 mice exhibited less ROS-induced DNA damage than WT mice after I/R ( Supplementary Fig. 5a ). In addition, the myocardial oxidized glutathione/reduced glutathione (GSSG/GSH) ratio, an indicator of intracellular redox status, was significantly elevated in WT mice but not in Tg-DN-Lats2 mice ( Supplementary Fig. 5b ). The size of the myocardial infarct/area-at-risk (AAR), indicative of necrotic cell death, as well as the number of apoptotic TUNEL (terminal deoxynucleotidyl transferase dUTP nick end labeling)-positive cells were significantly smaller in Tg-DN-Lats2 than in WT mice ( Supplementary Fig. 6a,b ). Furthermore, the same phenotype was observed in mouse models with cardiac-specific deletion of lats2 (Lats2-CKO) ( Supplementary Fig. 7a,b ). When we further assessed cardiac I/R injury using ex vivo models, we noted a similar decrease in infarct size in Tg-DN-Lats2 mice ( Supplementary Fig. 8a ), which was accompanied by improved function during the recovery phase of reperfusion as assessed by left ventricular (LV) developed pressure ( Supplementary Fig. 8b ). In sum, these data provide strong evidence that activation of Hippo signalling mediates oxidative stress-induced injury during I/R. 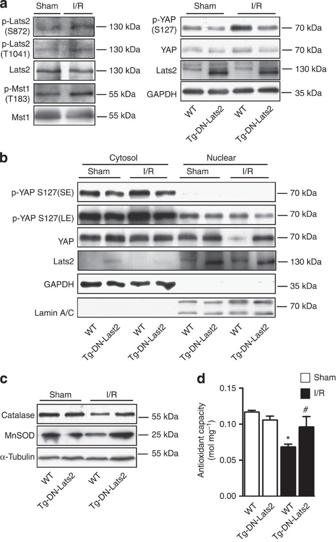Figure 4: Hippo activation stimulates oxidative stress in response to I/R. (a) Representative immunoblots indicating that I/R activated Hippo signalling. Left, WT mice were subjected to ischaemia for 45 min followed by 2 h of reperfusion. Sham and ischaemic area samples were used for immunoblot analysis for p-Lats2 (T1041 and S872), Lats2, p-Mst1 (Thr183) and Mst1. Right, Tg-DN-Lats2 and control WT mice were subjected to ischaemia for 45 min followed by 2 h of reperfusion. Sham and ischaemic area samples were used for immunoblot analysis for p-YAP (S127), YAP, Lats2 and GAPDH. The enhancement in YAP phosphorylation during I/R was attenuated in Tg-DN-Lats2, confirming that Lats2 activation was suppressed. (b) Tg-DN-Lats2 and control WT mice were subjected to ischaemia for 45 min followed by 2 h of reperfusion. The cytosolic and nuclear fractions of heart homogenates were prepared and subjected to immunoblot analysis of p-YAP (S127), YAP, Lats2, GAPDH and Lamin A/C (SE, short exposure; LE, long exposure). (c,d) Activation of Lats2 decreased antioxidant protein levels and enhanced oxidative stress during I/R. Tg-DN-Lats2 and control WT mice were subjected to ischaemia for 45 min followed by 24 h of reperfusion. (c) Sham and ischaemic area samples were used for immunoblot analysis for catalase, MnSOD, and α-tubulin. (d) The antioxidant capacity of the myocardium was examined (*P<0.05 versus WT/sham, #P<0.05 versus WT/I/R,n=4). Data are shown as mean±s.e.m.Pvalues were determined using one-way ANOVA followed by a Newman–Keuls comparison test. Figure 4: Hippo activation stimulates oxidative stress in response to I/R. ( a ) Representative immunoblots indicating that I/R activated Hippo signalling. Left, WT mice were subjected to ischaemia for 45 min followed by 2 h of reperfusion. Sham and ischaemic area samples were used for immunoblot analysis for p-Lats2 (T1041 and S872), Lats2, p-Mst1 (Thr183) and Mst1. Right, Tg-DN-Lats2 and control WT mice were subjected to ischaemia for 45 min followed by 2 h of reperfusion. Sham and ischaemic area samples were used for immunoblot analysis for p-YAP (S127), YAP, Lats2 and GAPDH. The enhancement in YAP phosphorylation during I/R was attenuated in Tg-DN-Lats2, confirming that Lats2 activation was suppressed. ( b ) Tg-DN-Lats2 and control WT mice were subjected to ischaemia for 45 min followed by 2 h of reperfusion. The cytosolic and nuclear fractions of heart homogenates were prepared and subjected to immunoblot analysis of p-YAP (S127), YAP, Lats2, GAPDH and Lamin A/C (SE, short exposure; LE, long exposure). ( c , d ) Activation of Lats2 decreased antioxidant protein levels and enhanced oxidative stress during I/R. Tg-DN-Lats2 and control WT mice were subjected to ischaemia for 45 min followed by 24 h of reperfusion. ( c ) Sham and ischaemic area samples were used for immunoblot analysis for catalase, MnSOD, and α-tubulin. ( d ) The antioxidant capacity of the myocardium was examined (* P <0.05 versus WT/sham, # P <0.05 versus WT/I/R, n =4). Data are shown as mean±s.e.m. P values were determined using one-way ANOVA followed by a Newman–Keuls comparison test. Full size image Inhibition of the YAP-FoxO1 complex mediates I/R injury If YAP-FoxO1 complex activity is essential for mediating cell survival during I/R, suppression of this complex should abolish the protective effect in Tg-DN-Lats2 mice and reactivation of this complex should rescue WT mice from I/R injury. To test this hypothesis, ad-sh-FoxO1 was injected into the LV and, 5 days later, I/R was performed. The efficacy of adenovirus injection was confirmed by whole-heart β-galactosidase staining in mice injected with Ad-LacZ ( Supplementary Fig. 6c ). The efficacy of ad-sh-FoxO1 injection was confirmed by immunoblot ( Supplementary Fig. 6d ). Compared with injection of control shRNA adenovirus (ad-sh-con), injection of ad-sh-FoxO1 significantly increased infarct size in Tg-DN-Lats2 mice, to the same level as in WT mice ( Fig. 5a ). Knocking down FoxO1 also significantly increased apoptosis in Tg-DN-Lats2 in response to I/R ( Fig. 5b ). As YAP has a direct positive effect on the regulation of the FoxO1-mediated antioxidant response, whether exogenous expression of YAP could rescue myocardial damage induced by I/R was also examined. Adenovirus harbouring WT YAP or a constitutively activated YAP mutant (S127A) was injected into the myocardium 3 days before I/R ( Supplementary Fig. 6e ) and infarct size was examined. 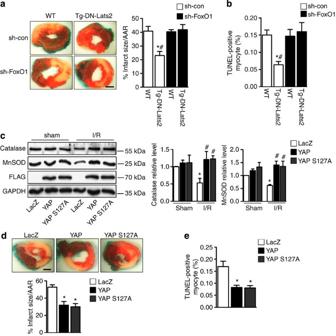Figure 5: Inhibition of Hippo protects against I/R injury. (a,b) Purified adenovirus (1 × 109opu) was administered by direct injection to the LV free wall (two sites, 25 μl per site) of Tg-DN-Lats2 and WT mice. I/R surgery was performed 5 days after injection. Mice were subjected to ischaemia for 45 min followed by 24 h of reperfusion. (a) Gross appearance of LV tissue sections after Alcian blue and triphenyltetrazolium chloride staining demonstrates that injection of ad-sh-FoxO1 abolished the protection observed in Tg-DN-Lats2 mice. Quantitative measurement of myocardial infarct area/AAR (% infarct size/AAR) was performed (*P<0.05 versus WT/sh-con, #P<0.05 versus Tg-DN-Lats2/sh-FoxO1,n=8). Scale bar, 1 mm. (b) LV myocardial sections were subjected to TUNEL staining. The number of TUNEL-positive myocytes was expressed as a percentage of total nuclei detected by DAPI staining (*P<0.05 versus WT/sh-con, #P<0.05 versus Tg-DN-Lats2/sh-FoxO1,n=5–8). (c–e) Purified adenovirus (1 × 109opu) was administered by direct injection to the LV free wall (two sites, 25 μl per site). I/R surgery was performed 3 days after injection. Mice were subjected to ischaemia for 30 min followed by 24 h of reperfusion. (c) Sham and ischaemic area samples were used for immunoblot analysis for catalase, MnSOD, and GAPDH. FLAG was also used to examine exogenous YAP gene expression. Statistical analyses of densitometric measurements of catalase and MnSOD are shown (*P<0.05 versus LacZ/sham, #P<0.05 versus LacZ/I/R,n=5). (d) Gross appearance of LV tissue sections after Alcian blue and triphenyltetrazolium chloride staining demonstrates that injection of YAP or YAP S127A decreased the infarct area. Quantitative measurement of myocardial infarct area/AAR (% infarct size/AAR) was performed (*P<0.05 versus LacZ,n=8). Scale bar, 1 mm. (e) LV myocardial sections were subjected to TUNEL staining. The number of TUNEL-positive myocytes was expressed as a percentage of total nuclei detected by DAPI staining (*P<0.05 versus LacZ,n=5–6). Data are shown as mean±s.e.m.Pvalues were determined using one-way ANOVA followed by a Newman–Keuls comparison test. Compared with injection of LacZ, both WT and S127A YAP significantly attenuated I/R-induced downregulation of catalase and MnSOD ( Figure 5c ) but did not affect endothelial nitric oxide synthase (eNOS) activity ( Supplementary Fig. 6f ). Furthermore, injection of adenovirus harbouring either WT or S127A YAP decreased the myocardial infarct size and cardiomyocyte apoptosis in response to I/R ( Fig. 5d,e ), suggesting that restoration of YAP-FoxO1 prevents cell death in response to oxidative stress induced by I/R. Figure 5: Inhibition of Hippo protects against I/R injury. ( a , b ) Purified adenovirus (1 × 10 9 opu) was administered by direct injection to the LV free wall (two sites, 25 μl per site) of Tg-DN-Lats2 and WT mice. I/R surgery was performed 5 days after injection. Mice were subjected to ischaemia for 45 min followed by 24 h of reperfusion. ( a ) Gross appearance of LV tissue sections after Alcian blue and triphenyltetrazolium chloride staining demonstrates that injection of ad-sh-FoxO1 abolished the protection observed in Tg-DN-Lats2 mice. Quantitative measurement of myocardial infarct area/AAR (% infarct size/AAR) was performed (* P <0.05 versus WT/sh-con, # P <0.05 versus Tg-DN-Lats2/sh-FoxO1, n =8). Scale bar, 1 mm. ( b ) LV myocardial sections were subjected to TUNEL staining. The number of TUNEL-positive myocytes was expressed as a percentage of total nuclei detected by DAPI staining (* P <0.05 versus WT/sh-con, # P <0.05 versus Tg-DN-Lats2/sh-FoxO1, n =5–8). ( c – e ) Purified adenovirus (1 × 10 9 opu) was administered by direct injection to the LV free wall (two sites, 25 μl per site). I/R surgery was performed 3 days after injection. Mice were subjected to ischaemia for 30 min followed by 24 h of reperfusion. ( c ) Sham and ischaemic area samples were used for immunoblot analysis for catalase, MnSOD, and GAPDH. FLAG was also used to examine exogenous YAP gene expression. Statistical analyses of densitometric measurements of catalase and MnSOD are shown (* P <0.05 versus LacZ/sham, # P <0.05 versus LacZ/I/R, n =5). ( d ) Gross appearance of LV tissue sections after Alcian blue and triphenyltetrazolium chloride staining demonstrates that injection of YAP or YAP S127A decreased the infarct area. Quantitative measurement of myocardial infarct area/AAR (% infarct size/AAR) was performed (* P <0.05 versus LacZ, n =8). Scale bar, 1 mm. ( e ) LV myocardial sections were subjected to TUNEL staining. The number of TUNEL-positive myocytes was expressed as a percentage of total nuclei detected by DAPI staining (* P <0.05 versus LacZ, n =5–6). Data are shown as mean±s.e.m. P values were determined using one-way ANOVA followed by a Newman–Keuls comparison test. Full size image Our results reveal that there is cross talk between the Hippo-YAP signalling pathway and FoxO1 in regulating cell death in response to oxidative stress ( Fig. 6 ). We discovered that YAP is a novel co-activator of FoxO1, and that the YAP-FoxO1 complex binds to the promoters of catalase and MnSOD, a step that is essential for expression of these antioxidant genes. Activation of the Hippo pathway during I/R inhibits the YAP-FoxO1 complex and suppresses expression of FoxO1 target genes, thereby enhancing oxidative stress and promoting cell death in cardiomoycytes. 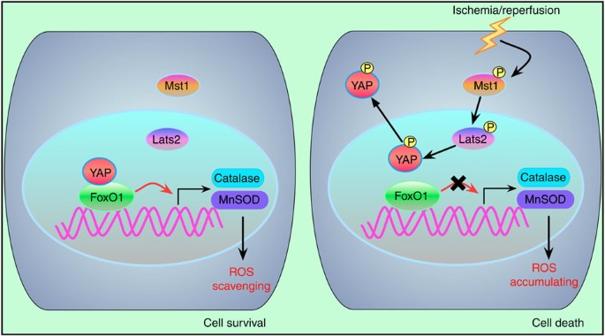Figure 6: A scheme of the cross talk between Hippo signalling and FoxO1. In cardiomyocytes, YAP and FoxO1 form a functional complex that mediates catalase and MnSOD expression. In response to I/R, activation of the Hippo signalling cascade induces YAP inactivation, which leads to antioxidant gene suppression, ROS accumulation and cell death. Figure 6: A scheme of the cross talk between Hippo signalling and FoxO1. In cardiomyocytes, YAP and FoxO1 form a functional complex that mediates catalase and MnSOD expression. In response to I/R, activation of the Hippo signalling cascade induces YAP inactivation, which leads to antioxidant gene suppression, ROS accumulation and cell death. Full size image FoxO1 activity is regulated by post-translational modifications, including phosphorylation and acetylation [15] . Akt phosphorylates FoxO1 at Thr 24 and Ser 256 , thereby inducing nuclear exit of FoxO1. However, overexpression of Lats2 induces nuclear exclusion of YAP without affecting either the activity of Akt or phosphorylation of FoxO1 at Thr 24 /Ser 256 ( Supplementary Figs 3d and 4d ). We have shown previously that overexpression of YAP in neonatal cardiomyocytes induces activation of Akt, thereby preventing cardiomyocyte death [12] . However, this was not accompanied by phosphorylation of FoxO1 at the Akt sites. These results suggest that YAP-mediated regulation of FoxO1 is independent of Akt-mediated phosphorylation. Deacetylation of FoxOs by Sirt1 also mediates cell survival during stress conditions [24] . We have shown previously that Sirt1 deacetylates FoxO1 and facilitates its nuclear translocation, thereby mediating a protective effect against I/R injury in the heart [25] . We here show that activation of Mst1 and Lats2 in response to I/R induces the nuclear exit of YAP, thereby negatively affecting the transcription of FoxO1 target genes, including catalase and MnSOD, even if FoxO1 is in the nucleus. Thus, although the activity of FoxO1 is regulated through multiple mechanisms, nuclear localization of endogenous YAP appears essential for transcriptional activation of FoxO1 in response to I/R, and this is critically regulated by the Hippo pathway. Mst1 has been show to phosphorylate FoxO3 that induces nuclear translocation of FoxO3 (ref. 13) [13] but inhibits its high-affinity DNA binding [26] , suggesting that this upstream component of the Hippo pathway can inhibit FoxOs independently of YAP. Here, however, we show that YAP, one of the terminal effectors of the Hippo pathway, also directly regulates FoxO1. Thus, the activity of FoxOs may be dually regulated by the components of the Hippo pathway; namely, activation of Mst1 and consequent suppression of YAP both negatively regulate transcription through FoxOs. At present, it remains unknown whether the regulation of FoxO by both upstream and downstream components of the Hippo pathway is stimulus-specific or coordinately regulates death and survival of cardiomyocytes. The transcriptional activity of FoxOs is also regulated by transcriptional co-factors. For example, the interaction between β-catenin and FoxO3 is important to prevent oxidative damage in cancer cell lines and control life span and the aging process in Caenorhabditis elegans [27] . In hepatocytes, the peroxisome proliferator-activated receptor-γ co-activator 1 interacts with FoxO1 and stimulates target gene expression to control glucose homeostasis [28] . Here we show that YAP-FoxO1 interaction is essential to mediate antioxidant gene expression in cardiomyocytes. The presence of multiple transcriptional regulators may allow FoxOs to tightly control expression of specific sets of target genes in a coordinated and stimulus-specific manner. TAZ shares ∼ 50% amino-acid sequence similarity with YAP. Both YAP and TAZ are negatively regulated by the Hippo pathway, bind to common transcription factors, including the Runx family and TEAD, and have redundant roles in several biological events, including tumorigenesis [29] , [30] , [31] . In the heart, both YAP and TAZ mediate embryonic heart growth and postnatal myocyte survival [8] , [9] , [12] . The fact that both YAP and TAZ interact with TBX5, a T-box transcription factor, suggests that YAP and TAZ may have overlapping roles during cardiac development [32] . However, they also have non-overlapping functions. For example, severe cardiac dysfunction results from αMHC-Cre (α myosin heavy chain-Cre recombinase)-mediated cardiac-specific deletion of YAP but not of TAZ [9] . On the other hand, genetic deletion of TAZ induces the development of renal cysts [33] . As downregulation of YAP inhibits FoxO1-mediated transcription, we speculate that TAZ may not compensate for the absence of YAP in cardiomyocytes. One key feature of highly proliferative cells is persistently enhanced ROS generation [34] , [35] . To overcome the generally pro-death actions of ROS, cancer cells develop adaptive mechanisms [36] , [37] , [38] that help the dividing cells escape premature senescence and apoptosis, as well as confer drug resistance to cancer cells [35] . Forkhead box transcription factors regulate both pro-survival genes and premature senescence [27] , [38] , suggesting the potential importance of FoxOs during tumour development and progression. In addition, increasing lines of evidence suggest that the Hippo pathway acts as a tumour suppressor in many organs. Loss-of-function mutations in the Hippo signalling pathway and hyperactivation of YAP have been found in multiple cancers [1] . Thus, it is tempting to speculate that regulation of antioxidant genes through the YAP-FoxO1 pathway may be a critical mechanism through which the Hippo pathway regulates tumorigenesis. In conclusion, our study shows a novel connection between the Hippo pathway and FoxO1 through YAP. As the Hippo pathway and FoxOs share many important functions, including regulation of growth, death and survival in cells, and regulation of stress resistance and life span in organisms, we speculate that the interaction between YAP and FoxO1 is a point of convergence that allows cells and organisms to precisely control important cellular functions through signals from these two major signalling pathways. Transgenic mice The generation of cardiac-specific dominant-negative lats2 transgenic mice on an FVB background (Tg-DN-Lats2) [11] , transgenic mice harbouring a floxed Yap1 allele [39] on C57BL/6 background, and transgenic mice harbouring a floxed lats2 allele [40] on C57BL/6 background has been previously described. Cardiac deletion was achieved by crossbreeding with α-MHC-Cre recombinase transgenic mice. Male mice aged 12–16 weeks were used for in vivo adenovirus injection and/or I/R surgery. All animal protocols were approved by the Institutional Animal Care and Use Committee of New Jersey Medical School, Rutgers Biomedical and Health Sciences. I/R surgery in vivo I/R was achieved by ligating the anterior descending branch of the left coronary artery (LAD) using an 8-0 prolene suture, with silicon tubing (1 mm OD) placed on top of the LAD, 2 mm below the border between the left atrium and LV. Ischaemia was confirmed by electrocardiogram (ECG) change (ST elevation). After occlusion for 45 min in mice of an FVB background and for 20–30 min in mice of a C57BL/6J background, the silicon tubing was removed to achieve reperfusion, and the rib space and overlying muscles were closed. Twenty-four hours after reperfusion, myocardial infarction was examined. To demarcate the ischaemic AAR, Alcian blue dye (1%) was perfused into the aorta and coronary arteries. Hearts were excised and LVs were sliced into 1-mm-thick cross-sections. The heart sections were then incubated with 1% triphenyltetrazolium chloride solution at 37 °C for 15 min. The infarct area (pale), the AAR (not blue) and the total LV area from both sides of each section were measured using Adobe Photoshop (Adobe Systems Inc.), and the values obtained were averaged. The percentage of area of infarction and AAR of each section were multiplied by the weight of the section and then totalled from all sections. AAR/LV and infarct area/AAR were expressed as percentages [25] . Langendorff-perfused mouse heart model of global I/R Mouse hearts were mounted on a Langendorff-type isolated heart perfusion system and subjected to retrograde coronary artery reperfusion with 37 °C oxygenated Krebs–Henseleit bicarbonate buffer (120 mM NaCl, 17 mM glucose, 25 mM NaHCO 3 , 5.9 mM KCl, 1.2 mM MgCl 2 , 2.5 mM CaCl 2 and 0.5 mM EDTA), pH 7.4, at a constant pressure of 80 mm Hg. A balloon filled with water was introduced into the LV through the mitral valve orifice and connected to a pressure transducer by a plastic tube primed with water. LV pressures and LV dP/dt were recorded with a strip chart recorder (Astro-Med, Inc.). The LV end-diastolic pressure was set at 4–10 mm Hg at the beginning of perfusion by adjusting the volume of the balloon in the LV, and the volume was kept constant throughout the experiment. After a 30-min equilibration period, the heart was subjected to 30 min of global ischaemia (at 37 °C) followed by 60 min of reperfusion [25] . Cell cultures H9C2 myoblast cells and Cos7 cells (American Type Culture Collection) were cultured at 37 °C in DMEM/F-12 (Life Technologies, Inc.) with 10% FBS. Primary cultures of ventricular cardiomyocytes were prepared from 1-day-old Crl: (WI) BR-Wistar rats (Harlan Laboratories). A cardiomyocyte-rich fraction was obtained by centrifugation through a discontinuous Percoll gradient. Cells were cultured in complete medium containing DMEM/F-12 supplemented with 5% horse serum, 4 μg ml −1 transferrin, 0.7 ng ml −1 sodium selenite (Life Technologies, Inc.), and 2 g l −1 bovine serum albumin (fraction V), 3 mM pyruvic acid, 15 mM HEPES, 100 μM ascorbic acid, 100 μg ml −1 ampicillin, 5 μg ml −1 linoleic acid and 100 μM 5-bromo-2′-deoxyuridine (Sigma). Myocytes were changed to serum-free medium 24 h before any experiment. Plasmids The mammalian expression vector for YAP (pHA-YAP) was generated by insertion of YAP cDNA into pcDNA3-HA, which contains a DNA fragment encoding the HA (5′-GGATCC TACCCATACGATGTTCCGGATTACGCTAGTCTC TAGTCGAC-3′; YPYDVPDYASL) tag inserted downstream of the CMV promoter of pcDNA3. Site-directed mutagenesis was performed to generate pHA-YAP (S94A) using the QuikChange mutagenesis kit (Agilent Technologies). The expression vector for YAP with deleted WW domain (pHA-YAPΔWW) was generated by PCR. The expression vector for YAP with N-terminal fragment (pHA-YAP N-terminal) was generated by insertion of YAP cDNA from amino acid 1-316 into pcDNA3-HA. Adenovirus constructs Adenovirus harbouring Lats2 and Mst1 has been described [11] . Adenoviruses harbouring shRNA for Lats2 (Ad-sh-Lats2), FoxO1 (Ad-sh-FoxO1) and YAP (Ad-sh-YAP) were generated as previously described using the following hairpin-forming oligos. For Lats2: 5′-GCAGGTTCTTCGACGACAA TTCAAGAGA TTGTCGTCGAAGAACCTGCCTTTTTT-3′; For FoxO1: 5′-CGCCAAACTCACTACACCAT TTCAAGAGA ATGGTGTAGTGAGTTTGGCTTTTTT-3′; For YAP: 5′-GGTCAGAGATACTTCTTAA TTCAAGAGA TTAAGAAGTATCTCTGACCTTTTTT-3′. The hairpin loop sequence is underlined. The adenoviruses used for in vivo injection were purified using the Adeno-X Maxi Purification Kit (Clontech). Antibodies Antibodies used for immunoblots were purchased from the indicated companies: catalase (1:3,000 dilution, no. ab1877) (Abcam), p-Akt (Ser473) (1:2,000 dilution, no. 9272), Akt (1:2,000 dilution, no. 9271), p-eNOS (Ser1177) (1:1,000 dilution, no. 9571), eNOS (1:1,000 dilution, no. 9586), p-FoxO1 (Thr24, Ser256) (1:1,000 dilution, nos. 9464 and 9461), FoxO3 (1:1,000 dilution, no. 9467), GAPDH (1:3,000 dilution, no. 2118), Histone H3 (1:500 dilution, no. 9715), Lamin A/C (1:5,000 dilution, no. 4777), p-Mst1 (Thr183) (1:1,000 dilution, no. 3681), p-YAP (Ser127) (1:1,000 dilution, no. 4911), YAP (1:2,000 dilution, no. 4912) (Cell Signaling Technology), FoxO1 (1:2,000 dilution, no. 1874-1) (Epitomics), α-tubulin (1:5,000 dilution, no. T-6199), FLAG (1:2,000 dilution, no. F3165) (Sigma), MnSOD (1:3,000 dilution, no. 611580), Mst1 (1:2,000 dilution, no. 611052) (BD Biosciences), and Lats2 (1:1,000 dilution, nos. ab54073 and A300-479A) (Abcam and Bethyl Laboratories). The p-Lats2 (S872 and T1041) (1:500 dilution) antibodies were generated as described [41] . Immunoblot analysis Heart homogenates or cell lysates were prepared using RIPA buffer containing 50 mM Tris (pH 7.4), 150 mM NaCl, 1% Triton X-100, 0.1% SDS, 1% deoxycholic acid, 1 mM EDTA, 1 mM Na 3 VO 4 , 1 mM NaF, 0.5 mM 4-(2-aminoethyl) benzenesulfonyl fluoride hydrochloride, 0.5 μg ml −1 aprotinin, and 0.5 μg ml −1 leupeptin. Equal amounts of protein (10–20 μg) were subjected to 10–15% SDS–PAGE. The nuclear and cytosolic fractions were prepared with NE-PER Nuclear and Cytoplasmic Extraction Reagents (Pierce). After proteins were transferred to a PVDF membrane, immunoblots were probed with the indicated antibodies. Full scans of all western blots and gels are supplied in Supplementary Fig. 9 . Immunoprecipitation Heart homogenates or cell lysates were prepared using a lysis buffer containing 50 mM Tris (pH 7.4), 150 mM NaCl, 1% Triton X-100 and 1 mM EDTA. The lysates were incubated with protein A agarose-immobilized antibody for 2 h at 4 °C. After immunoprecipitation, the immunocomplexes were washed with lysis buffer three times and eluted with 2 × SDS sample buffer. Immunocytochemistry Neonatal cardiomyocytes in four-well chambers were washed with phosphate-buffered saline (PBS) three times, fixed with 4% paraformaldehyde for 15 min, permeabilized in 0.3% Triton X-100 for 10 min and blocked with 3% bovine serum albumin for 1 h at room temperature. The following primary antibodies were used: Lats2 (1:200 dilution, no. ab54073) (Abcam), FoxO1 (1:100 dilution, no. 1874-1) (Epitomics), YAP (1:100 dilution, H00010413-M01) (Abnova) and α-actinin (1:400 dilution, A7811) (Sigma). Alexa Fluor 488 Dye- or Alexa Fluor 594 Dye-conjugated secondary antibody (Invitrogen) was used for detecting indirect fluorescence. Slides were mounted using a reagent containing 4′,6-diamidino-2-phenylindole (DAPI) (Vectashield) (Vector Laboratories Inc.). In situ PLA Neonatal cardiomyocytes were fixed, permeabilized and blocked as described as above. Heart sections were deparaffinized with xylene, rehydrated in graded alcohol concentrations, briefly washed in water and then antigen-unmasked using citrate buffer and blocked in 5% goat serum in PBST for 1 h. In situ PLA experiments were performed as described previously [42] , [43] . Incubation with primary antibodies (Rabbit FoxO1 and Mouse YAP in blocking solution) was performed at room temperature for 2 h. Cells or heart sections were washed for three times for 5 min in PBS plus 0.1% Tween 20. The protein–protein interaction between FoxO1 and YAP was detected with secondary proximity probes (Rabbit-PLUS and Mouse-MINUS) (Olink Biosciences AB). The secondary proximity probes were incubated for 1 h at 37 °C. Cells were washed once for 5 min in 10 mM Tris-HCl (pH 7.5) plus 0.1% Tween 20 at 37 °C, then twice for 5 min in PBS plus 0.1% Tween 20. All subsequent steps were performed according to the Duolink proximity ligation assay detection kit protocol (Olink Biosciences AB). Immunohistochemistry for 8-OHdG staining Anti-8-OHdG antibody (Oxis International Inc.) was diluted to 7.5 μg ml −1 in PBS and applied to tissue sections for 2 h at room temperature. The immunohistochemistry experiment was performed using the ImmunoCruz staining system (streptavidin–biotin peroxidase method; Santa Cruz Biotechnology), and sections were counterstained with hematoxylin. X-gal staining Heart tissues were fixed for 1 h in 0.1 M phosphate buffer (pH 7.3) supplemented with 5 mM EGTA, 2 mM MgCl 2 and 0.2% glutaraldehyde (Sigma). Fixed samples were washed three times for 15 min with 0.1 M phosphate buffer (pH 7.3) supplemented with 2 mM MgCl 2 , 0.01% Na deoxycholate and 0.02% NP-40 and then incubated in staining buffer containing 0.1 M phosphate buffer (pH 7.3), 2 mM MgCl 2 , 5 mM potassium ferrocyanide, 5 mM potassium ferricyanide, 0.01% Na deoxycholate, 0.02% NP-40 and X-gal at a final concentration of 1 mg ml −1 overnight at 37 °C. Detection of oxidative stress Fresh heart tissues were dissected and incubated in a Krebs/HEPES buffer containing 5 μM lucigenin. After 15 min of equilibration, counts were obtained every minute for the next 5 min in a luminometer. The O 2 − level was presented as chemiluminescence units normalized by tissue weight. For H 2 O 2 production, heart sections were incubated with Amplex Red (10 μM) for 30 min at 37 °C. The Amplex assay was performed according to the supplier’s protocol (Molecular Probes). Tissue homogenates were prepared using 5% metaphosphoric acid. The tissue level of GSSG/GSH was determined using the Bioxytech GSH/GSSG-412 kit (Oxis International Inc.). The antioxidant capacity of heart homogenates was determined using an antioxidant assay kit according to the supplier’s instructions (Cayman Chemical). RT–PCR and quantitative PCR Total RNA was isolated from neonatal cardiomyocytes using TRIzol (Invitrogen) and first-strand cDNA was synthesized using the ThermoScript RT-PCR system (Invitrogen). Quantitative PCR was carried out using a DNA Engine Opticon 2 system (Bio-Rad) and iQ SYBR Green Supermix (Bio-Rad). Catalase and MnSOD mRNA levels were analysed using specific primers. Values were standardized using β-actin. Quantitative PCR primers: catalase: forward: 5′-CCTCCTCGTTCAAGATGTGGTTT-3′, reverse: 5′-CCTTTGCCTTGGAGTATCTGGTAATA-3′; MnSOD: forward: 5′-CAACTCAGGTTGCTCTTCA-3′, reverse: 5′-CGACCTTGCTCCTTATTGA-3′; β-actin forward: 5′-AGGCCAACCGTGAAAAGATG-3′, reverse: 5′-ACCAGAGGCATACAGGGACAA-3′. CellTiter-Blue assay Cell viability was measured by CellTiter-Blue (CTB) assays (Promega). In brief, cardiomyocytes (1 × 10 5 per 100 μl) were seeded onto 96-well dishes. After 24 h, the cells were transduced with the indicated adenovirus. After transduction, myocytes were incubated with or without H 2 O 2 treatment. Viable cell numbers were measured by the CTB assay. The CTB assays were performed according to the supplier’s protocol. Transient transfection and luciferase assays Cells were plated on 12-well plates and transfected with 1 μg of the indicated luciferase vectors using Fugene 6. Total DNA quantity was kept constant. Six hours after transfection, the cells were washed and transduced with the indicated adenovirus. The cells were lysed with Passive Lysis Buffer, and the transcriptional activity was determined using a luciferase assay system (Promega). In vitro kinase assay Active Lats2 recombinant protein (10 ng) (Signal Chem) was incubated with 1 μg myc-FoxO1 recombinant protein (OriGene) in a kinase assay buffer containing 25 mM MOPS (pH 7.2), 12.5 mM β-glycerolphosphate, 25 mM MgCl 2 , 5 mM EGTA, 2 mM EDTA and 0.25 mM DTT. The reaction was initiated by adding [γ- 32 P] ATP (PerkinElmer) and was incubated for 30 min at 30 °C. The reaction was terminated by the addition of 2 × SDS sample buffer. Samples were separated by SDS–PAGE and the dried gel was subjected to autoradiography. ChIP and sequential ChIP H9C2 myoblasts were treated with 1% formaldehyde for 10 min to cross-link proteins and chromatin. The reaction was stopped by adding 0.125 M glycine for 5 min. Cells were washed with cold PBS twice. Cells were then resuspended in 1 ml ChIP lysis buffer (20 mM Tris–HCl (pH 8.0), 85 mM KCl, 0.5% NP-40) for 10 min at 4 °C and centrifuged at 5,000 r.p.m. to pellet the nuclei. The cell nuclei were resuspended in 400 μl nuclei lysis buffer (50 mM Tris-HCl (pH 8.0), 10 mM EDTA and 1% SDS) and then subjected to sonication five times for 30 s with 30 s intervals. Purified chromatin was analysed on a 1% agarose gel to determine the shearing efficiency. As a control, normal IgG was used as a replacement for YAP or FoxO1 antibody (Santa Cruz Biotechnology). For sequential ChIP, sheared chromatin was first immunoprecipitated with FoxO1, followed by elution and a second immunoprecipitation using the YAP antibody. The ChIP procedure was performed as in the supplier’s protocol (Active Motif). ChIP-PCR primers: Catalase promoter-DBE1: forward: 5′-GGTGGACTATTGACAGTGTTGGG-3′, reverse: 5′-CGCCATCCAGTTATTTACTCAGG-3′; catalase promoter-DBE2: forward: 5′-ACCAAATAAATAAGCAAAGTGAG-3′, reverse: 5′-GAAACTCTAGAAGGGACAGGATT-3′; MnSOD promoter-DBE1: forward: 5′-TCATGGCCACTATGCCTCAA-3′, reverse: 5′-TCTCAGCTGTGTCCTCTTCC-3′; MnSOD promoter-DBE2: forward: 5′-CCTCTTGTTTATTACATCAAGATTG-3′, reverse: 5′-CTGGTTGTCAACTTGACTATATC-3′. Statistical analysis All values are expressed as mean±s.e.m. Statistical analysis between groups was conducted by unpaired Student’s t -test or one-way analysis of variance (ANOVA) followed by a Newman–Keuls comparison test. Values of P <0.05 were considered to be significant. How to cite this article: Shao, D. et al. A functional interaction between hippo-YAP signalling and FoxO1 mediates the oxidative stress response. Nat. Commun. 5:3315 doi: 10.1038/ncomms4315 (2014).